Improving lithium–sulphur batteries through spatial control of sulphur species deposition on a hybrid electrode surface Lithium–sulphur batteries are attractive owing to their high theoretical energy density and reasonable kinetics. Despite the success of trapping soluble polysulphides in a matrix with high surface area, spatial control of solid-state sulphur and lithium sulphide species deposition as a critical aspect has not been demonstrated. Herein, we show a clear visual evidence that these solid species deposit preferentially onto tin-doped indium oxide instead of carbon during electrochemical charge/discharge of soluble polysuphides. To incorporate this concept of spatial control into more practical battery electrodes, we further prepare carbon nanofibers with tin-doped indium oxide nanoparticles decorating the surface as hybrid three-dimensional electrodes to maximize the number of deposition sites. With 12.5 μl of 5 M Li 2 S 8 as the catholyte and a rate of C/5, we can reach the theoretical limit of Li 2 S 8 capacity ~\n1,470 mAh g −1 (sulphur weight) under the loading of hybrid electrode only at 4.3 mg cm −2 . High-energy batteries have recently attracted great interest owing to the needs of energy storage in portable electronics, vehicle electrification and grid-scale stationary storage [1] . Sulphur is an abundant material available at large scale and low cost as the side product of petroleum and mineral refining, which makes it attractive for low-cost and high-energy Li–S batteries [1] , [2] , [3] , [4] . During the discharge of Li–S batteries, solid S cathodes go through a series of soluble polysulphide species (Li 2 S 8 , Li 2 S 6 and Li 2 S 4 ) and become solid Li 2 S 2 and Li 2 S [5] , [6] . During charging, Li 2 S 2 and Li 2 S are converted back to S via soluble polysulphide intermediates [7] , [8] . The dissolution of polysulphides in the electrolyte leads to the shuttle effect and uncontrolled deposition of S, Li 2 S 2 and Li 2 S, which is believed to be the main reason for low Coulombic efficiency and rapid capacity fade in Li–S batteries [6] , [8] , [9] . To address the issue of soluble polysulphides, one strategy is to trap soluble polysulphides inside porous conductive materials in cathodes. Exciting progress has recently been made in trapping polysulphide species in high surface area carbon [10] , oxide and polymer [11] , [12] , [13] , in hollow structures [14] , [15] , [16] and with binders [17] , [18] , [19] . The pioneering work by the Nazar et al. [1] on mesoporous carbon particles to encapsulate sulphur demonstrated the relatively high capacity of about 1,000 mAh g −1 for 20 cycles [10] . Other materials for trapping polysulphides to improve the performance include porous carbon spheres [20] , hollow carbon spheres [14] , hollow carbon nanofibers [15] , graphene oxides [21] , metal oxide particles [22] , metal-organic framework particles [11] , microporous carbon paper [23] and conductive polymers [13] , [24] . Although these conductive matrix-encapsulated sulphur cathodes have shown high specific capacities during the initial cycles, subsequent cycles usually show rapid capacity decay. Recently, recognizing the coupling effect of polysulphide dissolution and large volume expansion has led to excellent cycle life up to 1,000 cycles based on the S-TiO 2 yolk shell nanoparticles and hollow S nanoparticles capped by polymer shells, which have predesigned empty space to accommodate volume expansion without fracturing the shell materials [25] , [26] . Another promising approach, based on the different chemical bonding nature of S (nonpolar) and Li x S (polar), is to design bifunctional binders to trap polysulphides [18] , [27] . Despite exciting progress of trapping polysulphides, all these studies also show that there is still at least 10–20% sulphur loss as polysulphides into the electrolyte [10] , [25] , and thus it is very challenging to completely encapsulate all the S species [28] . Indeed, some studies indicate that Li–S batteries work through a dissolution-precipitation mechanism in order to have reversible charge/discharge, and it is necessary to have at least some soluble polysulphides [6] , [29] , [30] . The direct solid-state transformation between S and Li 2 S is kinetically too slow at room temperature [31] . Interestingly, it has been demonstrated that the dissolved polysulphides can form a stable solid electrolyte interphase (SEI) on the surface of lithium metal to suppress lithium dendrite growth [28] , [32] . Therefore, it seems necessary to develop another complementary strategy by recognizing that at least some soluble polysulphides exist in the electrolyte. Different from the previous sulphur encapsulation strategy, we turn our attention to spatial control of solid-state charge/discharge products in the cathode in order not to lose the activity of some dissolved S species. There are three issues to be considered on the deposition of S species: the uncontrolled random deposition of S or Li x S on limited surface area of electrodes could lead to the formation of large agglomerates that are electrochemically inactive [8] , [29] , [33] ; the slow redox kinetics of polysulphides on the surface of certain electrodes could result in the low utilization of sulphur during charge and discharge [34] ; and solid S species might bind weakly and detach away from the electrode surface and thus become inactive [27] . To address these issues related to the deposition of S species, the electrode surface in a Li–S battery should be able to control the deposition of polysulphides and have strong binding with the deposited sulphur species. The traditional carbon electrode with a nonpolar surface shows little affinity for the polysulphide deposition. In comparison, conductive tin-doped indium oxide (ITO), electrical conductivity up to ~\n10 4 S cm −1 , exhibits a hydrophilic surface, which is attractive for addressing the polysulphide deposition issues. Herein, an ITO pattern is introduced onto the electrode to improve the Li–S battery performance via the spatially controlled polysulphide deposition. The model study of the deposition of polysulphides From the recent theoretical understanding of the strong binding affinity of polysulphides, Li 2 S 2 and Li 2 S with polar surfaces [18] , [27] , we devised a model system for the spatial control of S species deposition using the coexistence of polar and nonpolar electrode surfaces by creating a regularly patterned ITO glassy carbon planar electrode ( Fig. 1a ). ITO glassy carbon-patterned hybrid electrodes were fabricated by sputtering 100-nm-thick ITO through a copper grid mask onto a glassy carbon substrate, resulting in 60 μm × 60 μm ITO squares separated by 15-μm-wide carbon lines. To demonstrate spatially controlled deposition, the ITO-C electrode was assembled as a cathode collector with Li metal as the anode and 2 M (the concentration based on sulphur) Li 2 S 8 polysulphide solution as the catholyte. Soluble polysulphide instead of solid-state S or Li 2 S was used as the starting S source since the random distribution of lithium polysulphide on the electrode ( Supplementary Fig. 1 ) does not interfere with subsequent characterization of the location of solid deposition products. The cell was first discharged to 1.7 V and kept at this voltage until the discharge current decreased to 1 μA cm −2 . Scanning electron microscopy (SEM) and energy dispersive X-ray spectroscopy (EDX) elemental analysis were used to identify the spatial distribution of discharge products on the electrodes. 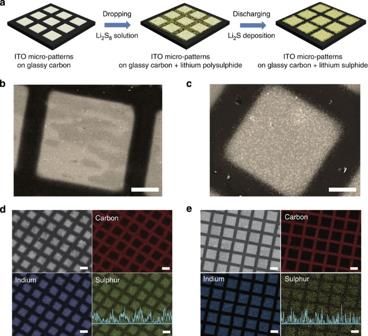Figure 1: Model system to demonstrate the strong bonding between polysulphides and ITO and preferred deposition of polysulphides on ITO. (a) Schematic illustration of the fabrication of polysulphide-ITO micropattern glassy carbon cathode to show the nature of polysulphide deposition. (b,c) The corresponding SEM images of a fresh ITO micropattern, and LixS-ITO micropattern, respectively. Scale bar, 20 μm. (d,e) EDX mapping of ITO glassy carbon electrode after discharging to 1.7 V and charging to 2.6 V, respectively, showing clearly patterned distributions of carbon (red), indium (blue) and sulphur (green). Scale bar, 50 μm. Figure 1: Model system to demonstrate the strong bonding between polysulphides and ITO and preferred deposition of polysulphides on ITO. ( a ) Schematic illustration of the fabrication of polysulphide-ITO micropattern glassy carbon cathode to show the nature of polysulphide deposition. ( b , c ) The corresponding SEM images of a fresh ITO micropattern, and Li x S-ITO micropattern, respectively. Scale bar, 20 μm. ( d , e ) EDX mapping of ITO glassy carbon electrode after discharging to 1.7 V and charging to 2.6 V, respectively, showing clearly patterned distributions of carbon (red), indium (blue) and sulphur (green). Scale bar, 50 μm. Full size image The surface of the as-fabricated ITO glassy carbon hybrid electrode is smooth with ITO patches being bright and C being dark in the SEM images, respectively ( Fig. 1b ). After discharge, the ITO pattern has many particles on the surface while the C surface still looks smooth, suggesting that the discharge solid products are mainly on the ITO surface ( Fig. 1c ). The magnified SEM image ( Supplementary Fig. 2 ) further shows the vertical platelet-like structures of these nanoparticles on the ITO surface. We mapped out the relevant elemental (C, S and In) distribution with EDX in SEM ( Fig. 1d ). Lithium is too light to be detected in EDX. Figure 1d (top left) shows an SEM image of the mapped electrode surface after discharge. The sulphur map (green, bottom right) overlays very well with the indium map (blue, bottom left) while there is only little sulphur on carbon map (red, top right), suggesting the discharged Li x S species are mostly deposited on the ITO surface. The line scan of the sulphur signal across the sample displayed sharp variations in signal intensity consistent with the patterned morphologies and high contrast between the ITO and the carbon surfaces. The effect of changing the width and spacing of the ITO patterns on the spatial distribution of Li x S species was studied as well ( Supplementary Fig. 3 and Supplementary Note 1 ). The results indicate that the selective deposition of Li x S species onto ITO is effective even on patterns with width and spacing on the order of 1 μm. To further demonstrate the formation of Li x S after discharging to 1.7 V and the strong bonding between the formed Li x S and ITO, we used the X-ray photoelectron spectroscopy (XPS) to analyse the deposition products on glassy carbon and ITO-coated glassy carbon electrodes, respectively. As shown in Supplementary Fig. 4 , the binding energy peaks around 160 eV of the S 2p spectra indicate the formation of Li x S on the electrodes after discharging to 1.7 V [35] , [36] . The Li 1s spectra ( Supplementary Fig. 5 ) show a 0.5-eV red shift of the Li 1s -binding energy of Li x S on the ITO-carbon surface compared with that of Li x S on the carbon surface, which indicates a strong bonding interaction between Li x S and ITO [27] , [35] . The ITO glassy carbon hybrid electrode after charge was investigated as well. The conversion of polysulphide to sulphur in the charging process was confirmed by Raman spectroscopy ( Supplementary Fig. 6 ). Figure 1e shows an SEM image and EDX mapping of an ITO glassy carbon hybrid electrode after one cycle of discharging to 1.7 V and then charging to 2.6 V. Although the nonpolar charging product (sulphur) has higher affinity with carbon compared with ITO [18] , [22] , [27] , the S elemental mapping still matched with the ITO mapping, indicating that more sulphur attaches to the ITO surface than to the carbon surface. This patterning distribution of sulphur after charging is related to the strong bonding between polysulphides and ITO. During the charging process, the polysulphides are intermediates that prefer to be adsorbed on ITO surface. Only during the last stage (~\n2.4 V) of the charging process the polysulphides are transformed into sulphur. However, the transformation occurs quite quickly and the sulphur is in the solid state, which largely suppresses the diffusion of nonpolar sulphur to the nonpolar carbon surface. In addition, varying the charge current density did not affect the spatial deposition of lithium polysulphides on patterned electrodes ( Supplementary Note 2 ). At a high current density of 200 μA cm −2 , preferential sulphur deposition onto ITO was still observed after the direct charging of polysulphides ( Supplementary Fig. 7 ). Furthermore, the Li x S-ITO micropatterns can still be observed after 20 charge/discharge cycles and ending at the discharged Li x S state ( Supplementary Fig. 8 ), indicating the strong adsorption of polysulphides on the ITO surface during charge/discharge cycling. Free-standing ITO-C nanofiber hybrid electrode fabrication To incorporate the ITO-C hybrid interface design into practical Li–S batteries, we fabricated free-standing carbon nanofiber nonwoven mats decorated with ITO nanoparticles as a binder-free sulphur cathode. The key point of the fabrication process for ITO-carbon hybrid nanofibers is to construct core-shell nanofibers formed by a phase-separated solution by co-electrospining [37] , [38] , [39] . In our fabrication process, a dimethyl formamide solution containing four components (polyacrylonitrile (PAN), polypyrrolidone (PVP), In(NO 3 ) 3 and SnCl 4 ) was first prepared, in which In 3+ and Sn 4+ serve as the ITO precursors coordinated with PVP, forming a separated phase from PAN due to the different viscosities of PVP and PAN [39] . By co-electrospinning this solution, the PAN with higher viscosity acts as a discontinuous (droplet) phase to form the core of the nanofiber, whereas the PVP-ITO precursor acts as the continuous (surrounding) phase to form the shell of nanofiber ( Fig. 2a ) [37] . The electrospun PAN/PVP-ITO core/shell nanofibers were calcined in air at 300 °C for 4 h, which yielded nanocrystalline ITO nuclei assembled on the surface of oxidized PAN nanofibers due to the thermal decomposition of PVP. Further, the oxidized PAN nanofibers were carbonized under Ar at 800 °C for 2 h to form ITO nanoparticle-decorated conducting carbon nanofibers. As a control sample, carbon nanofibers were prepared by the same procedure except without adding ITO precursor into the electrospinning solution. ITO-C hybrid nanofibers and carbon nanofibers were characterized by transmission electron microscope (TEM) and SEM to reveal their nanostructures. Both fibres have well-defined one-dimensional nanostructures with diameters around 180 nm±20 nm ( Fig. 2b,e ; Supplementary Fig. 9a,c ). In contrast to the smooth surface of carbon nanofibers, many small nanoparticles are attached to the surface of ITO-C nanofibers ( Fig. 2c,f ; Supplementary Fig. 9b,d ). High-resolution TEM images ( Fig. 2d,g ) show that the nanoparticles on the ITO-carbon nanofibers are highly crystalline and the carbon in both nanofibers is amorphous. The number density of ITO nanoparticles on the carbon nanofibers is 12±2 per 50 nm × 50 nm square. The average distance between ITO particles is ~\n10 nm. Compared with the microscale ITO patterns shown in the planar glassy carbon electrode, the polysulphides diffusion at the nanoscale space among these ITO nanoparticles will facilitate the spatially controlled deposition of polysulphides. The size of ITO nanoparticles is in the range of 3~\n20 nm. The ITO nanoparticles on the surface of the carbon nanofibers was further characterized by EDX ( Supplementary Fig. 10 ) and identified as the cubic phase by powder X-ray diffraction ( Supplementary Fig. 11 ). Lattice fringes with 2.92 Å d-spacing in Fig. 2d correspond to the (222) crystal planes of cubic phase ITO. 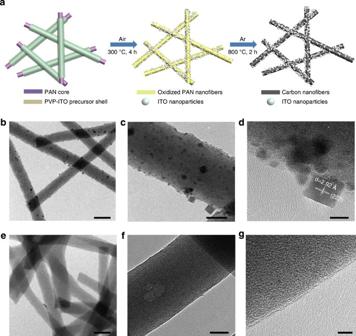Figure 2: Fabrication procedure and TEM images of ITO-C hybrid and carbon nanofibers. (a) Schematic illustration of the fabrication of ITO-C hybrid nanofibers. The core/shell PAN/PVP-ITO precursor nanofibers were prepared by single-nozzle co-electrospinning. With subsequent two-step calcination treatments, the ITO nanoparticles-decorated carbon nanofibers were obtained. (b,c) TEM images of ITO-C hybrid nanofibers showing well-defined one-dimensional nanostructures and many nanoparticles on the surface of the nanofibers. (d) High-resolution TEM image of ITO-C nanofibers showing crystalline ITO nanoparticles on the amorphous carbon nanofibers. (e–g) TEM images of carbon nanofibers for comparison with ITO-C nanofibers. (b,e) Scale bar, 200 nm. (c,f) Scale bar, 50 nm. (d,g) Scale bar, 10 nm. Figure 2: Fabrication procedure and TEM images of ITO-C hybrid and carbon nanofibers. ( a ) Schematic illustration of the fabrication of ITO-C hybrid nanofibers. The core/shell PAN/PVP-ITO precursor nanofibers were prepared by single-nozzle co-electrospinning. With subsequent two-step calcination treatments, the ITO nanoparticles-decorated carbon nanofibers were obtained. ( b , c ) TEM images of ITO-C hybrid nanofibers showing well-defined one-dimensional nanostructures and many nanoparticles on the surface of the nanofibers. ( d ) High-resolution TEM image of ITO-C nanofibers showing crystalline ITO nanoparticles on the amorphous carbon nanofibers. ( e – g ) TEM images of carbon nanofibers for comparison with ITO-C nanofibers. ( b , e ) Scale bar, 200 nm. ( c , f ) Scale bar, 50 nm. ( d , g ) Scale bar, 10 nm. Full size image The discharge of polysulphides onto ITO-C hybrid nanofibers To study the effect of ITO nanoparticles on the electrochemical performance of Li–S batteries, coin cells with Li metal as the counter/reference electrode and 12.5 μl of 5 M polysulphides (Li 2 S 8 ) as a catholyte were fabricated. The obtained free-standing electrospun nanofiber mats were punched into discs with diameter of 1.11 cm and were directly used as current collectors ( Supplementary Fig. 12 ). It is worth noting that these electrospun nanofiber electrodes provide a conductive surface for polysulphide deposition during the charge/discharge process of Li–S batteries. Also, the empty space between nanofibers can accommodate the volume change that occurs between S and Li 2 S [40] . And more importantly, the ITO nanoparticles distributed on nanofiber electrodes can enable the spatial control of polysulphide deposition on electrodes to improve the utilization efficiency of active materials. The typical mass loading of sulphur in the electrode was 2 mg cm −2 , and specific capacities were calculated based on sulphur only. For a fair comparison, the mass of the chosen electrodes was the same (3 mg, ~\n90 μm thick). The electrochemical impedance analysis of as-fabricated Li–S cells before cycling ( Supplementary Fig. 13 ) shows a lower charge transfer resistance of ITO-C electrode compared with that of carbon nanofiber electrode, which indicates a faster redox kinetics of polysulphides on the surface of the ITO-C hybrid electrode [41] . The initial discharge and charge voltage profiles at C/5 (1 C=1,673 mA g −1 ) of these electrodes are shown in Fig. 3a . At the beginning of discharge, the voltage decreased linearly to around 2.1 V without the typical first plateau of Li–S batteries. The linear decrease of voltage from 2.3 to 2.1 V corresponds to the conversion from long-chain polysulphides (Li 2 S 8 ) to short-chain polysulphides (Li 2 S 4 ). Both ITO-C nanofiber electrode and C nanofiber alone show similar specific capacity of 190 mAh g −1 (theoretically 209 mAh g −1 ) between 2.3 and 2.1 V, indicating that conversion of Li 2 S 8 to Li 2 S 4 has similar high efficiency. The typical second voltage plateau at around 2.1 V, which is also found in conventional Li–S batteries, corresponds to the phase change from liquid Li 2 S 4 to solid Li 2 S 2 or Li 2 S. For the charge process, the voltage profile is the same as that of typical Li–S batteries owing to the total phase change from Li 2 S 2 or Li 2 S to sulphur. Impressively, the initial discharge capacity of the ITO-C hybrid nanofiber electrode can reach 1,279 mAh g −1 , more than twice that of the carbon electrode (620 mAh g −1 ). 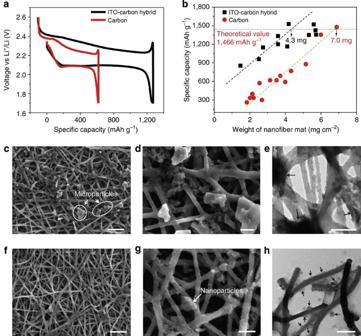Figure 3: Initial discharge of polysulphide and LixS deposition on the electrospun nanofiber electrodes. (a) Initial discharge/charge voltage profiles at a C/5 current rate of ITO-C and carbon nanofiber electrode, respectively. (b) Plot of initial discharge capacities of ITO-C and carbon nanofiber electrodes at C/5 current rate as the function of the mass of the used electrodes. (c–e) SEM image, magnified SEM image and TEM image of a carbon nanofiber electrode after discharge showing the microparticles formed on the nanofiber electrode. (f–h) SEM image, magnified SEM image and TEM image of ITO-C nanofiber electrode after discharge showing the nanoparticles formed on the nanofiber electrode. Arrows were used to mark the particles on the nanofibers. (c,f) Scale bar, 2 μm. (d,e,g,h) Scale bar, 500 nm. Note that the capacity enhancement of ITO-C compared with that of the carbon electrode mainly comes from the voltage plateau at around 2.1 V. Figure 3: Initial discharge of polysulphide and Li x S deposition on the electrospun nanofiber electrodes. ( a ) Initial discharge/charge voltage profiles at a C/5 current rate of ITO-C and carbon nanofiber electrode, respectively. ( b ) Plot of initial discharge capacities of ITO-C and carbon nanofiber electrodes at C/5 current rate as the function of the mass of the used electrodes. ( c – e ) SEM image, magnified SEM image and TEM image of a carbon nanofiber electrode after discharge showing the microparticles formed on the nanofiber electrode. ( f – h ) SEM image, magnified SEM image and TEM image of ITO-C nanofiber electrode after discharge showing the nanoparticles formed on the nanofiber electrode. Arrows were used to mark the particles on the nanofibers. ( c , f ) Scale bar, 2 μm. ( d , e , g , h ) Scale bar, 500 nm. Full size image Since the capacity of Li–S batteries largely depends on the conductive surface area (and thus the mass of electrode with the same diameters), we measured the discharge capacities of the same volume (12.5 μl) of 5 M Li 2 S 8 solution with a series of carbon and ITO-C nanofiber electrodes with different masses at C/5 to further show the enhanced effect of ITO nanoparticles on initial discharge capacity of Li–S batteries. As shown in Fig. 3b , the capacities of both electrodes increased with their weight, which is consistent with the increase of conductive surface area. In the range of 2–5 mg, the capacities of ITO-C electrodes are almost twice as that of carbon electrodes of the same weight. To achieve the full discharge of polysulphides with a capacity of 1,466 mAh g −1 (from Li 2 S 8 to Li 2 S), the weight of ITO-C nanofiber electrodes is 4.3 mg, much lighter than that of the carbon nanofiber electrode (7 mg), indicating that the ITO nanoparticles on carbon nanofibers enhanced the solid-state Li 2 S 2 and Li 2 S deposition efficiency on the electrode. The Li x S deposition on ITO-C hybrid nanofibers The nanofiber electrodes after initial discharge were investigated to reveal the spatially controlled deposition of polysulphides on the ITO-C hybrid electrode. As shown in Fig. 3c,f , many large particles up to 2 μm in diameter appeared on the carbon nanofiber mat electrode but only much smaller particles were found on the ITO-C hybrid nanofiber electrode after the initial discharge. The magnified SEM images ( Fig. 3d ) further show that the several microparticles were attached on the smooth surface of carbon nanofiber electrodes. For comparison, there are many nanoparticles (tens of nanometres in diameter) on the surface of the ITO-C nanofibers ( Fig. 3g ). These results suggest that ITO-C nanofibers provide much more deposition sites for Li x S than do the C nanofibers alone. TEM images ( Fig. 3e,h ) further show that there are more nanoparticles attached on the surface of the ITO-C hybrid electrode than on the carbon electrode. The particles on the electrodes were identified as sulphide species by the EDX spectra and line scans on these nanofibers ( Supplementary Fig. 14 ). The sulphur elemental distribution on the ITO-C hybrid nanofiber electrode is more homogeneous than that on the carbon nanofiber electrode ( Supplementary Fig. 15 ). As demonstrated in the planar ITO glassy carbon-patterned hybrid electrode, the ITO nanoparticles attached to the surface of carbon nanofibers act as ‘anchors’ to locate the polysulphides on the surface of the electrode promoting their redox kinetics and deposition efficiency. The ITO-C hybrid electrodes also provide both polar (ITO) and nonpolar (C) platform to facilitate binding of solid Li x S and S species on electrodes. The cycling performance of ITO-C hybrid nanofiber electrodes The fabricated batteries based on nanofiber electrodes also displayed excellent cycling stabilities, effectively resolving the fast capacity fading commonly observed in Li–S batteries with high-concentration polysulphides as starting materials [34] , [42] . The typical charge/discharge voltage profile of the fabricated cell in the following cycles ( Supplementary Fig. 16 ) indicates the complete reversible conversion between sulphur and lithium sulphide in the cell. As shown in Fig. 4a , the ITO-C hybrid nanofiber electrode (3 mg of electrode with 12.5 μl of 5 M Li 2 S 8 ) delivers reversible specific capacity above 1,000 mAh g −1 after 300 cycles at C/5 with a capacity decay of 0.04% per cycle. The carbon nanofiber electrode with the same electrode mass and mass loading of Li 2 S 8 , on the other hand, exhibits a lower specific capacity around 700 mAh g −1 . The average Coulombic efficiencies for ITO-C and carbon electrodes over 200 cycles are 99.8% and 99.6%, respectively. The stable reversible specific capacities of nanofiber electrodes are attributed to the accommodation of volume change provided by the empty space among nanofibers and the robustness of the nonwoven mat structure of the nanofiber electrode in avoiding structural failure during cycling. It is worth noting that the specific capacity of the cell dropped at first and then gradually increased in the first 50 cycles. This variation was caused by the redistribution of polysulphides on the nanofiber network and the reactivation of lithium sulphides formed on the lithium anode. In our cell fabrication ( Supplementary Fig. 17 and Supplementary Note 3 ), the polysulphide was directly dropped on the nanofiber mat that would lead to its inhomogeneous distribution in the nanofiber network. During the charge/discharge cycling, the polysulphides tend to form a homogenous distribution in the whole nanofiber network. In addition, polysulphides are highly reactive towards the fresh lithium metal owing to the lack of SEI protection during the first charge process. With the formation of SEI on the lithium metal surface in the following cycles, some reduced polysulphides were reactivated and diffused back into the nanofiber electrode. The cycling stability was also supported by testing for sulphur dissolution in the electrolyte after charge using inductively coupled plasma-optical emission spectroscopy ( Supplementary Fig. 18 and Supplementary Note 4 ). The percentage of dissolved sulphur after cycling at the charged state is in the range of 20~\n35% indicating the good cycling reversibility of the cell. 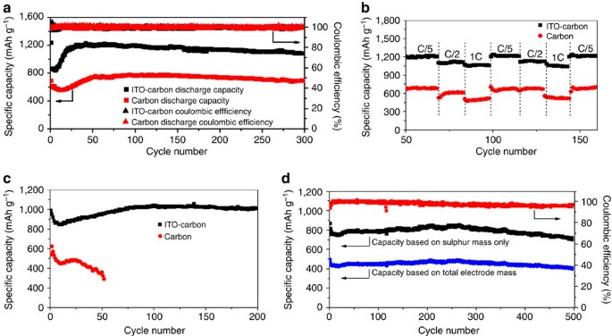Figure 4: Cycling performance of Li–S batteries using nanofiber mats as electrodes. (a) Discharge capacity and Coulombic efficiency of ITO-C hybrid nanofiber electrodes over 300 cycles at C/5 in comparison with carbon nanofiber electrodes. (b) Specific capacity of cells based on ITO-C nanofiber electrodes at C/5 (0.669 mA), C/2 (1.67 mA) and 1C (3.34 mA), respectively, in comparison with carbon nanofiber electrodes. (c) Discharge capacity of ITO-C hybrid nanofiber electrodes with high sulphur mass loading (4 mg cm−2) over 200 cycles at C/5. (d) Discharge capacity and Coulombic efficiency of ITO-C hybrid nanofiber electrode loaded with solid sulphur and polysulphides over 500 cycles at C/5. Figure 4b shows the excellent rate capability of these cells, further demonstrating the robustness of nanofiber electrodes. The ITO-C hybrid electrode delivers reversible specific capacity values of 1,200 mAh g −1 , 1,100 mAh g −1 and 1,050 mAh g −1 at C/5, C/2 and 1C, respectively. The carbon nanofiber electrode shows reversible specific capacity of 680 mAh g −1 , 600 mAh g −1 and 490 mAh g −1 at C/5, C/2 and 1C, respectively. With different charge/discharge rates, the ITO-C hybrid electrode showed more stable specific capacity with cycling than that of the carbon nanofiber electrode, indicating better stability of the ITO-C hybrid electrode. Figure 4: Cycling performance of Li–S batteries using nanofiber mats as electrodes. ( a ) Discharge capacity and Coulombic efficiency of ITO-C hybrid nanofiber electrodes over 300 cycles at C/5 in comparison with carbon nanofiber electrodes. ( b ) Specific capacity of cells based on ITO-C nanofiber electrodes at C/5 (0.669 mA), C/2 (1.67 mA) and 1C (3.34 mA), respectively, in comparison with carbon nanofiber electrodes. ( c ) Discharge capacity of ITO-C hybrid nanofiber electrodes with high sulphur mass loading (4 mg cm −2 ) over 200 cycles at C/5. ( d ) Discharge capacity and Coulombic efficiency of ITO-C hybrid nanofiber electrode loaded with solid sulphur and polysulphides over 500 cycles at C/5. Full size image The mass loading of sulphur on the ITO-C hybrid electrode is further increased to 4 mg cm −2 (57 wt.% based on the electrode mass of 3 mg) while retaining high specific capacity and outstanding cycling performance. As shown in Fig. 4c , the reversible capacity of the cell was maintained at 1,034 mAh g −1 over 200 cycles at C/5 without any capacity decay. The areal capacity of this cell is up to 4 mAh cm −2 , which is comparable to commercial battery values. As a comparison, the cell using carbon nanofibers as an electrode showed low capacity and fast capacity fading, further demonstrating the advantage of ITO-C hybrid electrode in high mass loading Li–S batteries. Although the cells using polysulphide solution (5 M) as the catholytes exhibited high specific capacity, the volumetric energy density of such a cell is as low as 461 Wh l −1 ( Supplementary Note 5 ). To increase the volumetric energy density (up to 829 Wh l −1 based on theoretical calculation in Supplementary Note 6 ), we replaced a fraction of polysulphides with solid sulphur. Figure 4d shows the cycling performance at C/5 of the cell using 2 mg of solid sulphur and 12.5 μl of 5 M Li 2 S 8 (2 mg of equivalent sulphur) as the catholyte. A reversible specific capacity of 710 mAh g −1 was obtained with capacity decay of 0.036% per cycle and an average Coulombic efficiency of 97.2% over 500 cycles. This means that the volumetric energy density of the Li–S cell can be enhanced by adding solid sulphur into the electrode without impairing the cycling stability. The sulphur-patterning distribution on the ITO-C planar electrode has shown the clear visual evidence, for the first time, to prove the spatial control of solid-state discharge products via a hybrid electrode design. On the basis of the patterned deposition of polysulphides, the strong bonding between polysulphides and the ITO surface provided an alternative route to enhance the performance of Li–S batteries through controlling nucleation and deposition of solid S/Li 2 S species. This ITO-C hybrid interface design is significantly different from the previously reported work on metal oxide additives to suppress the diffusion of polysulphides, such as mesoporous silica [12] , titania [22] , alumina [43] , Mg 0.6 Ni 0.4 O (ref. 44 ) and metal-organic frameworks [11] , as we demonstrate the importance of engineering the ITO-C hybrid interface in facilitating the polysulphide deposition. By constructing ITO nanoparticle-decorated carbon nanofiber mat via electrospinning, this hybrid electrode surface design has been realized in a practical Li–S battery exhibiting high mass loading and long-life cycling capabilities. The favourable bonding interaction between polysulphides and ITO nanoparticles on carbon nanofibers promoted the nucleation, reduction and deposition of the solid-state Li 2 S 2 and Li 2 S ( Supplementary Fig. 19 and Supplementary Note 7 ), which suggests that the spatial control of polysulphide deposition was realized in the ITO-C hybrid nanofiber electrodes for practical battery applications. However, several opening issues should be addressed for using this hybrid electrode design in practical batteries such as the density of the hybrid electrode, relatively high price of ITO and using lithium metal as the anode. In our fabricated ITO-carbon nanofiber hybrid electrode, the backbone of the electrode is constructed by the carbon nanofiber and the ITO nanoparticles were only attached on its surface. The usage efficiency of ITO nanoparticles were largely improved due to their exposure on the surface of the carbon nanofibers. In this case, the amount of ITO (a few percentages) used in our hybrid electrode is very low compared with the carbon component. Thus, the density and the cost of the ITO-carbon hybrid electrode are close to that of the pure carbon electrode. To address the issues of using lithium metal anode, two potential approaches have been proposed for Li–S batteries. One route is using a protection layer on the lithium metal surface to avoid the ‘shuttle effect’ of polysulphides and the lithium metal dendrite growth [32] , [45] . The other route is to replace the lithium metal by the pre-lithiated silicon/graphite [46] . In our present cells, in the presence of LiNO 3 and lithium polysulphides, a relatively stable SEI is formed on the surface of the lithium metal anode, which to a limited degree suppressed the ‘shuttle effect’ of polysulphides and the dendrite growth on the lithium metal surface [32] , [35] . As shown in Supplementary Fig. 20 , the S, C, N and O elements were detected by XPS on the surface of the lithium anode after cycling. The S 2p spectra show that some polysulphides were reduced to lithium sulphide species (Li 2 S and Li 2 S 2 ) on the anode surface. The existence of S–O (Li 2 SO 4 and Li 2 S 2 O 3 ) and –CO 2 Li (CH 3 CO 2 Li and CH 3 OCO 2 Li) indicates that LiNO 3 plays an important role as an oxidizing agent in the formation of the SEI. Meanwhile, the decomposition products of the electrolyte (RCH 2 OLi and ROLi) and the reduced products of LiNO 3 (LiN x O y and Li 2 N 2 O 2 ) also contributed to the formation of SEI. Furthermore, the smooth surface of the lithium metal anode after 20 cycles ( Supplementary Fig. 21 ) indicates that the lithium dendrites were suppressed by the SEI formed on the lithium metal surface. Our results show that the formed SEI layer is a promising protection layer to achieve the long cycling capability of Li–S batteries ( Supplementary Note 8 ). However, we note that the Li metal anode safety issue is not solved and requires future study. In summary, we proposed the ITO-carbon hybrid interface design to understand the spatially controlled deposition of polysulphides on the surface of electrodes and demonstrated its feasibility to improve the performance of Li–S batteries. The polar surface of ITO nanoparticles on the carbon nanofibers can enhance the redox kinetics of polysulphides and mediate the deposition of polysulphides, and the growth of Li x S on the electrode. This rational strategy for electrode surface modification will open a new direction to fabricate high-performance advanced Li–S and Li-air batteries. Lithium polysulphide (Li 2 S 8 ) solution preparation The Li 2 S 8 solution was prepared by dissolving a desired amount of stoichiometric S and Li 2 S in 1,3-dioxolane (DOL)/1,2-dimethoxyethane (DME) solution (1:1 in volume) with the addition of LiNO 3 additive (5 wt.%). For the typical preparation of 5 M Li 2 S 8 solution, 0.56 g of sulphur and 0.115 g of Li 2 S were added to 4 ml of DOL (2 ml)/DME (2 ml) mixed solution. The obtained suspension was stirred and heated at 80 °C overnight to yield red-brown Li 2 S 8 solution. Li x S-ITO glassy carbon micropattern fabrication Copper TEM grids (200 mesh) were attached on the surface of glassy carbon as the mask for ITO micropattern fabrication. A thin layer (100 nm) of ITO was sputtered (AJA ORION sputtering system) on the copper grid-covered glassy carbon to form the ITO micropatterns on the glassy carbon. The fabricated micropatterned ITO glassy carbon was used as the hybrid electrode to assemble the Li–S pouch cell. Twenty microlitres of 2 M polysulphide solution (Li 2 S 8 ) was placed on the ITO glassy carbon and then a piece of the separator with the electrolyte was put on the ITO glassy carbon. A piece of lithium metal was attached to the separator to form the ITO glassy carbon/separator/lithium metal sandwich structure, which was put into a pouch with an aluminium ribbon connecting to the glassy carbon and a copper ribbon connecting to the lithium metal, and sealed to form a pouch cell. The obtained cell was discharged to 1.7 V with a current of 20 μA cm −2 and kept at 1.7 V until the discharge current decreased to 1 μA cm −2 , or the cell was discharged to 1.7 V and then charged to 2.6 V until the charge current decreased to 1 μA cm −2 . After the discharge or charge, the cells were disassembled and the ITO glassy carbon electrodes were washed with DOL and dried for further characterization. The assembly and disassembly processes were carried out in an argon-filled glove box. ITO-carbon hybrid nanofiber electrode preparation PAN (0.5 g) ( M w =150,000), 0.5 g of PVP ( M w =1,300,000), 0.225 g of In(NO 3 ) 3 × H 2 O and 0.0176, g of SnCl 4 ·5H 2 O were dissolved in 10 ml of dimethyl formamide by heating at 80 °C with constant stirring. The freshly prepared solution was electrospun using a conventional electrospinning setup with the following parameters: 16 KV of static electric voltage, 12 cm of air gap distance and 0.3 ml h −1 flow rate of solution. A carbon paper (8 cm × 8 cm) was used as a collection substrate. After 3 h of electrospinning, the formed nanofiber mat on the carbon paper was transferred into a box furnace, heated up to 300 °C and held at this temperature for 4 h to oxidize the PAN nanofibers. After the oxidization process, the nanofiber mat was self-detached from the carbon paper forming the free-standing film. The free-standing oxidized PAN nanofiber films were further carbonized under an argon atmosphere at 800 °C for 2 h to generate ITO-C hybrid nanofiber films. Electrochemistry To evaluate the electrochemical performance of nanofiber electrodes, 2023-type coin cells (MTI Corporation) were assembled using lithium metals as the counter/reference electrode. The obtained free-standing electrospun nanofiber mats were punched into disks with diameter of 1.11 cm and directly used as current collector-free electrodes. The 5-M Li 2 S 8 solution was used as the active material. For a sulphur mass loading of 2 mg, 12.5 μl of 5 M Li 2 S 8 solution was added into a cell. The electrolyte was a freshly prepared solution of lithium bis(trifluoromethanesulphonyl)imide (1 M) in 1:1 v/v 1,2-DME and 1,3-DOL containing LiNO 3 (1 wt%). Electrolyte (20 μl) was added in one cell. The separator used is Celgard polyethylene separator with the thickness of 25 μm. 2032-type coin cells were assembled in an argon-filled glove box and galvanostatic cycling of cells was carried out using a 96-channel battery tester (Arbin Instruments). Characterization An FEI XL30 Sirion SEM with an field emission gun (FEG) source and energy dispersive spectroscopy detector was used for SEM characterization. An FEI Tecnai G2 F20 X-TWIN TEM was used for TEM characterization. XPS data were collected by an SSI S-Probe XPS Spectrometer and a PHI Versa Probe Scanning XPS Microprobe. XRD was done with a PANalytical X'Pert PRO X-ray diffraction system. Inductively coupled plasma-optical emission spectroscopy data were collected by the Thermo Scientific ICAP 6300 Duo View Spectrometer. The Raman spectra were collected by a Horiba Jobin Yvon Raman equipped with a 532-nm laser. How to cite this article: Yao, H. et al. Improving lithium–sulphur batteries through spatial control of sulphur species deposition on hybrid electrode surface. Nat. Commun. 5:3943 doi: 10.1038/ncomms4943 (2014).